Gekko japonicusgenome reveals evolution of adhesive toe pads and tail regeneration Reptiles are the most morphologically and physiologically diverse tetrapods, and have undergone 300 million years of adaptive evolution. Within the reptilian tetrapods, geckos possess several interesting features, including the ability to regenerate autotomized tails and to climb on smooth surfaces. Here we sequence the genome of Gekko japonicus (Schlegel’s Japanese Gecko) and investigate genetic elements related to its physiology. We obtain a draft G. japonicus genome sequence of 2.55 Gb and annotated 22,487 genes. Comparative genomic analysis reveals specific gene family expansions or reductions that are associated with the formation of adhesive setae, nocturnal vision and tail regeneration, as well as the diversification of olfactory sensation. The obtained genomic data provide robust genetic evidence of adaptive evolution in reptiles. Reptiles diverged from early tetrapods in the late Carboniferous period approximately 310–320 million years ago (Myr ago) [1] . Since then, these ancient amniotes have spread across the world and adopted diverse morphologies and habitats (aquatic and terrestrial) [2] . More than 10,000 reptile species have been documented and they are classified into the following four orders: Crocodilia, Testudines, Squamata and Sphenodontia [3] . Squamate reptiles represent the most diverse radiation of terrestrial vertebrates and are traditionally split into two major clades, Iguania and Scleroglossa [3] , [4] . The latter clade includes the terrestrial Gekkonidae, which consists of ∼ 1,450 species in 118 genera and comprises 25% of all described lizard species [5] . Geckos have evolved in a terrestrial niche, where selective pressure [6] has resulted in traits such as small body size, agility and nocturnal habits. Most gecko species possess adhesive toe pads, which enable them to capture live food more easily, and flee from their predators by scaling vertical or even inverted surfaces [7] . This ability is due to the presence of setae, microscopic hair-like outgrowths of the superficial layer of the subdigital epidermis, which comprise the primary components of the adhesive apparatus [7] , [8] . The most interesting and physiologically significant trait in geckos is their ability to voluntarily shed or autotomize their tails to escape from attack, they then regenerate a new tail [9] . Given these interesting characteristics, geckos have been used in studies on regenerative processes, and their adhesive mechanism has been examined for the development of bio-inspired technologies [10] . The availability of genome sequence data would significantly contribute to deciphering the evolutionary events related to lineage-specific anatomical adaptations. To date, the genomes of several reptilian species, including species from Squamata reptiles ( Anolis carolinensis , Python molurus bivittatus and Ophiophagus hannah ), Crocodylia reptiles ( Alligator sinensis , Alligator mississippiensis , Gavialis gangeticus and Crocodylus porosus ) and Testudines reptiles ( Chelonia mydas , Pelodiscus sinensis and Chrysemys picta bellii ) have been successfully sequenced [11] , [12] , [13] , [14] , [15] . These results have filled the genomic gap between amphibians and birds by providing genomic information on a wide variety of morphologically and physiologically distinct species. However, genomic data from the species comprising the family Gekkonidae, which is an important clade of Lepidosauria and one of the earliest branches off the squamata phylogenetic tree, have not yet been acquired. In this study, the genome of G. japonicus (Schlegel’s Japanese Gecko) is sequenced and annotated, which provides valuable insights into the adaptive evolution of geckos as well as the genomic basis of their characteristic traits. For example, our data reveals that the expansion of β-keratin gene family is essential to the clinging ability of G. japonicus , and the evolution of the opsin gene is correlated with its visual adaptation. Moreover, some positive selected genes (PSGs) potentially involved in the tail regeneration are identified as well. In addition, developing a genomic resource associated with geckos is helpful in understanding the evolutionary history of Lepidosauria. Sequencing and annotation of the G. japonicus genome The genome of an adult male G. japonicus was sequenced and assembled ( Supplementary Figs 1–3 and Tables 1–3 ). The draft genome sequence of G. japonicus was 2.55 Gb in size, ∼ 50% larger than that of Anolis carolinensis , a lizard that belongs to the Iguania of Squamata, making it the largest sequenced genome to date among all reptiles with available genome data [11] , [12] , [13] , [14] . The assembly quality was assessed using 10 fosmid clones and RNA-Seq data ( Supplementary Fig. 4 and Tables 4–6 ). Repeated elements were annotated using Repeat Masker program [16] . The repeats comprised 48.94% of the genome, and most were transposable elements, making up 48.02% of the assembly ( Supplementary Fig. 5 and Tables 7 and 8 ). The GC content in G. japonicus genome was about 45.5%, which is slightly higher than in genome of other amniotes (for example, Anolis. carolinensis , 40.3%; Gallus gallus , 41.5%; Homo sapiens , 40.8%). The GC content was primarily distributed in introns, the intergenic regions and CDS regions ( Supplementary Figs 6 and 7 ). Collectively, the above data indicate that the large genome size of G. japonicus may primarily result from the greater abundance of repeated sequences compared with other genomes, such as that of A. carolinensis ( Supplementary Tables 9–12 ). 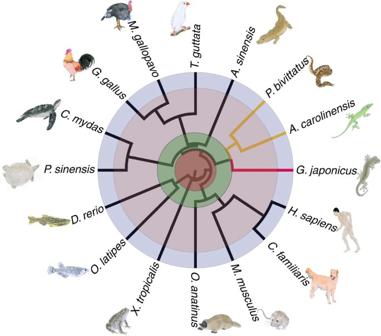Figure 1: Phylogenetic analysis of the whole-genomes of 6 reptilian species and 10 additional vertebrate species. The species in the phylogenetic tree includeDanio rerio(D. rerio),Xenopus tropicalis(X. tropicalis),Chelonia mydas(C. mydas),Pelodiscus sinensis(P. sinensis),Alligator sinensis(A. sinensis),Python molurus bivittatus(P. bivittatus),Anolis carolinensis(A. carolinensis),Gekko japonicus(G. japonicus),Taeniopygia guttata(T. guttata),Gallus gallus(G. gallus),Ornithorhynchus anatinus(O. anatinus),Canis familiaris(C. familiaris),Mus musculus(M. musculus),Homo sapiens(H. sapiens),Oryzias latipes(O. latipes) andMeleagris gallopavo(M. gallopavo). Before the Permian period is represented in brown. The Permian period to the Triassic period is represented in green. The Triassic period to the Paleogene period is represented in purple. The Paleogene period to the present is represented in blue. A total of 22,487 coding regions and 1,302 non-coding RNAs were predicted in the G. japonicus genome ( Supplementary Tables 13–15 ), and ∼ 95.08% of the coding regions were functionally annotated ( Supplementary Table 16 ). Then, the orthologous and paralogous genes were clustered and compared among different species background ( Supplementary Figs 8–10 and Tables 17 and 18 ). The data revealed that G. japonicus had 11,513 orthologous gene pairs compared with A. carolinensis , and the mean identity reached up to 72.37% ( Supplementary Fig. 9 and Table 18 ). A comparison of gene data among four reptiles ( G. japonicus , An. carolinensis , Al. sinensis and C. mydas ) revealed ∼ 13,478 orthologous gene families in total, of which 7,546 were shared by four species, 1,240 were specific to G. japonicus , 798 were specific to An. carolinensis , 911 were specific to Al. sinensis and 673 were specific to C. mydas ( Supplementary Fig. 10 ). These species-specific unique orthologous may be involved in lineage-specific adaptations. Evolutionary analysis of the G. japonicus genome We assessed evolutionary relationships among morphologically and ecologically diverse reptiles by constructing a phylogenetic tree using the whole-genomes of 6 reptilian species and 10 other vertebrates. The results support the view that the species of Gekkota diverged early from the group containing Anolis and Python ∼ 200 Myr ago [17] , when Gondwanaland separated from Laurasia [18] . This time period is earlier than previous reported [19] , but later than the divergence of Sphenodon [20] . A. carolinensis clusters with P. bivittatus rather than with G. japonicus , indicating that A. carolinensis and P. bivittatus have a much closer genetic relationship, even though P. bivittatus and G. japonicus have traditionally been classified as scleroglossans [4] . The phylogenetic tree shows that the crocodilian lineage diverged from chelonian about 250 Myr ago and clusters in the same clade with birds ( Fig. 1 ). A second phylogenetic tree constructed with conserved housekeeping proteins shows consistent results with these findings ( Supplementary Fig. 11 ). The cladogram of whole-genomes clearly shows the evolutionary relationships among these selected amniotes, and the whole genome resource will reduce the ambiguities of phylogeny data when assessed by previous methods based on morphological characteristics or few genes [17] , [19] . Figure 1: Phylogenetic analysis of the whole-genomes of 6 reptilian species and 10 additional vertebrate species. The species in the phylogenetic tree include Danio rerio ( D. rerio ), Xenopus tropicalis ( X. tropicalis ), Chelonia mydas ( C. mydas ), Pelodiscus sinensis ( P. sinensis ), Alligator sinensis ( A. sinensis ), Python molurus bivittatus ( P. bivittatus ), Anolis carolinensis ( A. carolinensis ), Gekko japonicus ( G. japonicus ), Taeniopygia guttata ( T. guttata ), Gallus gallus ( G. gallus ), Ornithorhynchus anatinus ( O. anatinu s), Canis familiaris ( C. familiaris ), Mus musculus ( M. musculus ), Homo sapiens ( H. sapiens ), Oryzias latipes ( O. latipes ) and Meleagris gallopavo ( M. gallopavo ). Before the Permian period is represented in brown. The Permian period to the Triassic period is represented in green. The Triassic period to the Paleogene period is represented in purple. The Paleogene period to the present is represented in blue. Full size image Adaptive evolution of setae β-keratins in G. japonicus The emergence of novel lineage-specific morphological features is always accompanied with genes duplications and diversions. A prominent example is the large-scale duplication of β-keratin genes that has been crucial to the evolution of scales, claws, beaks and feathers in reptiles and birds. The emergence of setae in geckos also resulted from the duplication and diversion of β-keratin genes. The clinging ability of geckos depends primarily on spade-like adhesive setae [21] . Previous reports have indicated that setae are comprised of a corneous material largely made of β-keratins of 8–22 kDa, with cysteine-rich proteins located in setae/spatula, and glycine-rich proteins in the β-layer of epidermis [22] . In addition, β-keratins have high isoelectric points with positive charges that enhance Van der Waals adhesion in the setae. These physicochemical properties indicate that β-keratin proteins are key to the clinging ability of setae [23] . To investigate whether the β-keratin genes are associated with varying adhesive ability in different reptile species, we retrieved the β-keratin genes from the genomes of G. japonicus , An. carolinensis and Al. sinensis , which possess branched setae, unbranched setae and no setae, respectively. Our analysis showed that the β-keratin gene families have undergone major expansion corresponding with adhesive ability ( Supplementary Table 19 ). G. japonicus , An. carolinensis and Al. sinensis contain 71, 23 and 2 β-keratin genes, respectively ( Fig. 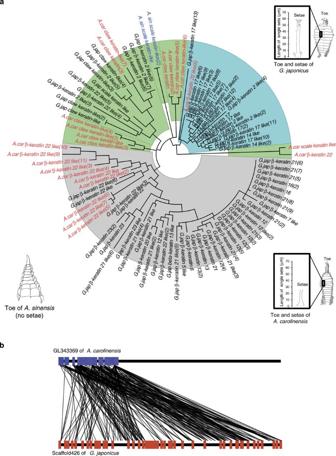Figure 2: Phylogenetic tree ofβ-keratinfamilies fromG. japonicus,An. carolinensisandAl. sinensis. (a) Theβ-keratinsin black font belong toG. japonicus, those in red belong toAn. carolinensisand those in blue belong toAl. sinensis. Gene copy number is listed in parentheses. The green background denotes β-keratins in scales and claws. The grey background denotes β-keratins in setae. The blue background denotes β-keratins in digital scales and pad lamella for supporting setae. A schematic diagram of toe ofG. japonicus,An. carolinensisandAl. sinensis, which possess branched setae, unbranched setae and no setae are presented, respectively. The setae of geckoG. japonicusare∼60 μm in length, and that inAn. carolinensisis∼25 μm. (b) Synteny diagram ofβ-keratingenes inA. carolinensis(upper line: GL343369, blue: 23β-keratingenes) andG. japonicus(lower line: scaffold 426, red: 48β-keratins). 2 , Supplementary Table 20 ). The majority of the extensively expanded families in G. japonicus genome contained the setae β-keratins genes important for setae production. These β-keratin proteins are usually characterized with S-core box (SEVTIQPPPCTVVVPGPVLA), cysteine-rich and low-molecular weight ( ∼ 10 kDa), which had been investigated in Gekko gecko . In the G. japonicus genome, 35 setae β-keratins with featured S-core box were identified among all 71 β-keratins by aligning them with amino acid sequences of S-core box (sequence similarity ≥70%). Additional important features associated with the above β-keratins, such as cysteine content and molecular weight were summarized in Fig. 3a and Supplementary Table 20 . Furthermore, most setae β-keratins were clustered on a single scaffold (scaffold 426) of the G. japonicus assembly, suggesting regional duplication events. These genomic characteristics may be related to the need for vast abundance of proteins to create the large number of setae in G. japonicus . In the other two species, a total of 16 setae β-keratin genes were identified in the An. carolinensis genome, and no setae β-keratin genes were found in the Al. sinensis genome. This result suggested that β-keratin genes expansion is positively correlated with setae formation in the assessed species. To date the periods of setae β-keratin expansion in G. japonicus , we established a phylogenetic tree using 133 β-keratin protein sequences from several reptiles and birds [24] , and calculated the divergence value of the branch site in the tree. The timescale of β-keratin expansion was determined by reference to the timescale of divergence of scale and claw β-keratins in birds ( ∼ 156 Myr ago) and the period of feather keratins expansion (66–51 Myr ago) [25] , [26] . The results showed that setae β-keratins experienced twice expansions: one at 105–96 Myr ago and the other at 87–80 Myr ago ( Fig. 3b ). The expansion period of setae β-keratin genes proposed by this strategy was very close to the period of setae emergence in gecko indicated by fossil evidence [27] . Of course, the comparative analysis of β-keratin genes expansion is based on only three genomes, and it is not possible to conclude whether the patterns seen in the G. japonicus genome are unique to this species. Figure 2: Phylogenetic tree of β-keratin families from G. japonicus , An. carolinensis and Al. sinensis . ( a ) The β-keratins in black font belong to G. japonicus , those in red belong to An. carolinensis and those in blue belong to Al. sinensis . Gene copy number is listed in parentheses. The green background denotes β-keratins in scales and claws. The grey background denotes β-keratins in setae. The blue background denotes β-keratins in digital scales and pad lamella for supporting setae. A schematic diagram of toe of G. japonicus , An. carolinensis and Al. sinensis , which possess branched setae, unbranched setae and no setae are presented, respectively. The setae of gecko G. japonicus are ∼ 60 μm in length, and that in An. carolinensis is ∼ 25 μm. ( b ) Synteny diagram of β-keratin genes in A. carolinensis (upper line: GL343369, blue: 23 β-keratin genes) and G. japonicus (lower line: scaffold 426, red: 48 β-keratins ). 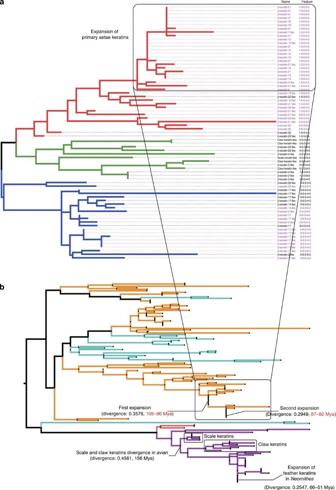Figure 3: Evolutionary analysis of setaeβ-keratins. (a) Phylogenetic tree ofβ-keratinsfromG. japonicus. The red branches represent β-keratins belonging to the primary components of setae, the blue branches represent the components in pad lamella for supporting setae and the green branches represent β-keratins in scales or claws. A total of 48β-keratins(purple font) are clustered in scaffold 426, of these 46 have a single exon. The combinatorial numbers following the keratin names indicate the following protein characteristics: 1: S-core box (SEVTIQPPPCTVVVPGPVLA, sequence similarity ≥70%, 35 proteins); 2: cysteine-rich (Cys >10%, 19 proteins); 3: glycine-rich (Gly >15%, 36 proteins); 4: isoelectric point (pI >7, 34 proteins); 5: molecular weight (Wt <15,000, 58 proteins); 0: none of the above.β-keratinsassociated with clinging ability have undergone extensive expansion and have higher isoelectric points. (b) Calculation of the expansion period for primary gecko setaeβ-keratinsusing protein sequences from 71β-keratinsofG. japonicas(orange), 23β-keratinsofAn. carolinensis(light blue), 2β-keratinsofAl. sinensisand 1β-keratin-like ofCrocodylus niloticus(pink), and 36β-keratinsassociated with bird’s claw, scale and feather (violet, including the following birds:Gallus gallus,Chlamydotis macqueenii,Opisthocomus hoazin,Mesitornis unicolor,Haliaeetus leucocephalus,Leptosomus discolor,Nestor notabilis,Chaetura pelagica,Pterocles gutturalis,Tinamus guttatus,Pygoscelis adeliae,Tauraco erythrolophus,Manacus vitellinus,Picoides pubescens,Mycteria americana,Cathartes auraandEurypyga helias). The divergence of scale and clawkeratinsoccurs in a birds ancestor∼156 Myr ago, and the featherkeratinsexpansion occurred in birds∼66 Myr ago.β-keratinsin setae ofG. japonicushave undergone two expansion periods: one approximately 105–96 Myr ago and the other approximately 87–80 Myr ago. Full size image Figure 3: Evolutionary analysis of setae β - keratins . ( a ) Phylogenetic tree of β-keratins from G. japonicus . The red branches represent β-keratins belonging to the primary components of setae, the blue branches represent the components in pad lamella for supporting setae and the green branches represent β-keratins in scales or claws. A total of 48 β-keratins (purple font) are clustered in scaffold 426, of these 46 have a single exon. The combinatorial numbers following the keratin names indicate the following protein characteristics: 1: S-core box (SEVTIQPPPCTVVVPGPVLA, sequence similarity ≥70%, 35 proteins); 2: cysteine-rich (Cys >10%, 19 proteins); 3: glycine-rich (Gly >15%, 36 proteins); 4: isoelectric point (pI >7, 34 proteins); 5: molecular weight (Wt <15,000, 58 proteins); 0: none of the above. β-keratins associated with clinging ability have undergone extensive expansion and have higher isoelectric points. ( b ) Calculation of the expansion period for primary gecko setae β-keratins using protein sequences from 71 β-keratins of G. japonicas (orange), 23 β-keratins of An. carolinensis (light blue), 2 β-keratins of Al. sinensis and 1 β-keratin- like of Crocodylus niloticus (pink), and 36 β-keratins associated with bird’s claw, scale and feather (violet, including the following birds: Gallus gallus , Chlamydotis macqueenii , Opisthocomus hoazin , Mesitornis unicolor , Haliaeetus leucocephalus , Leptosomus discolor , Nestor notabilis , Chaetura pelagica , Pterocles gutturalis , Tinamus guttatus , Pygoscelis adeliae , Tauraco erythrolophus , Manacus vitellinus , Picoides pubescens , Mycteria americana , Cathartes aura and Eurypyga helias ). The divergence of scale and claw keratins occurs in a birds ancestor ∼ 156 Myr ago, and the feather keratins expansion occurred in birds ∼ 66 Myr ago. β-keratins in setae of G. japonicus have undergone two expansion periods: one approximately 105–96 Myr ago and the other approximately 87–80 Myr ago. Full size image Nocturnal vision adaptation in G. japonicus As a nocturnal animal, G. japonicus possesses several sensory system characteristics, such as light sensitivity [28] , reduced colour vision, multifocal optical system, high olfaction [29] and special auditory senses [30] . Collectively, these features improve the ability of G. japonicus to catch prey, evade predators and communicate in low-light environments [28] . Vertebrate photoreceptor cells are categorized as rods and cones. Rods are responsible for dim-light vision, and cones for daylight and colour vision. Most geckos are nocturnal and possess retinas primarily made up of single and double cones [31] . A premise termed the transmutation theory, proposes that cones in nocturnal geckos were transformed from the cones of some ancestral diurnal lizard [32] . We assessed our genome data for evidence indicating how retinal pigment genes evolved during scotopic adaptation. The photosensitive molecules within photoreceptor cells consist of chromophore and opsin (protein moiety). The visual opsins are classified into five paralogs: rod pigments RH1 (rhodopsin), cone pigments RH2 ( RH1 -like), SWS1 (short wavelength-sensitive type 1), SWS2 ( SWS1 -like) and LWS / MWS (long wavelength-sensitive and middle wavelength-sensitive). We identified nine opsin genes in the genome of G. japonicus and 20 opsin genes in the genome of A. carolinensis ( Supplementary Tables 21 and 22 ), a diurnal lizard with typical tetra chromatic visual system. Our analysis revealed that A. carolinensis possessed a complete set of opsin paralogs, while G. japonicus had only three functional opsins : SWS1 , LWS and RH2 , all of which are usually found in cones ( Supplementary Table 22 ). In searching for the remaining two opsins, we were able to identify the rod pigment RH1 and the cone pigment SWS2 in G. japonicus , however, they were nonfunctional pseudogenes. The phylogenetic relationship between the opsins form different species is shown in Fig. 4b . We found that RH1 was more divergent between G. japonicus and A. carolinensis than was SWS2 , indicating that the loss of RH1 occurred earlier than that of SWS2 ( Fig. 4a ). These results were in agreement with the hypothesis that the ancestors of modern geckos are diurnal lizard without rod opsins [28] . These ancestral species later lost the cone opsin SWS2 , potentially as a partial adaptation towards nocturnal vision [33] . Our data provide, for the first time, the evidence of a RH1 deficiency at the genome level in nocturnal geckos. 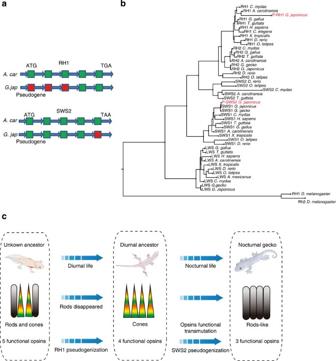Figure 4:Opsinsgenes in theG. japonicusgenome. (a) Analysis ofRH1andSWS2pseudogenes showed mutations in both initiation and termination codons. In addition, the exons ofRH1andSWS2inG. japonicuswere lost, incomplete or shifted in comparison with those inA. carolinensis. The green boxes indicate exons with similarity to those inA. carolinensis. The red boxes represent the lost exons. (b) Phylogenetic analysis ofopsingenes fromDrosophila melanogaster,Danio rerio,Oryzias latipes,Xenopus tropicalis,Chelonia mydas,Gallus gallus,Taeniopygia guttata,Anolis carolinensis,Gekko geckoandHomo sapiens. The pseudogenes inG. japonicus(P-RH1andP-SWS2) are indicated in red. (c)Opsinevolution inG. japonicusat genomic level agrees with observed evolutionary variation of retinal cell type and visual sense. Figure 4: Opsins genes in the G. japonicus genome. ( a ) Analysis of RH1 and SWS2 pseudogenes showed mutations in both initiation and termination codons. In addition, the exons of RH1 and SWS2 in G. japonicus were lost, incomplete or shifted in comparison with those in A. carolinensis . The green boxes indicate exons with similarity to those in A. carolinensis . The red boxes represent the lost exons. ( b ) Phylogenetic analysis of opsin genes from Drosophila melanogaster , Danio rerio , Oryzias latipes , Xenopus tropicalis , Chelonia mydas , Gallus gallus , Taeniopygia guttata , Anolis carolinensis , Gekko gecko and Homo sapiens . The pseudogenes in G. japonicus ( P-RH1 and P-SWS2 ) are indicated in red. ( c ) Opsin evolution in G. japonicus at genomic level agrees with observed evolutionary variation of retinal cell type and visual sense. Full size image These data lead to the question of what functional opsins are responsible for nocturnal vision in G. japonicus . Previous reports have suggested that opsin RH2 amino acid site 89 is an important functional determinant of rod and cone visual pigments [33] . Our comparative analysis indicated that RH2 in G. japonicus possesses the amino acid replacements F89C, which enables RH2 to have rod pigment-specific biochemical characteristics [32] , [33] , [34] ( Supplementary Table 23 ). Our results suggest a possible functional switch or compensatory change in cone pigment of gecko that allows them to receive more light. In conclusion, our results surrounding the evolution of opsin genes at genomic level support the hypothesis that nocturnal G. japonicus evolved from the diurnal ancestors. Furthermore, the pseudogenization and functional switch of opsins is concordant with the variation of retinal cell type, which includes the loss of rods and transformation of cones ( Fig. 4c ). One thing to note here is that the evolution pattern of opsin we proposed is based on genome data of few species. More data, including genomes of other related species, and phylogenetic analyses are necessary to test this hypothesis and to determine how and when particular changes occurred in the opsin families. Diversified olfaction of G. japonicus Improved survival in a low-light environment typically includes the evolution of more sensitive sense of smell to better obtain food and safety [35] . Our analysis of expanded gene families in 16 species revealed that G. japonicus had a significant expansion of olfactory receptor (OR) genes. OR genes are divided into Class I and Class II. The Class I genes encode odour receptors that detect molecules in water, and can be divided into the following sub-groups: α , β , ɛ , ζ and δ . The class II genes encode odour receptors that detect molecules in air, and only have a γ sub-group [36] . According to our gene family analysis, G. japonicus displayed more diversity of OR genes ( α- , β- and γ -ORs) than any of other assessed reptiles and more than even human ( α- , γ -ORs). Usually, a single air OR can only identify one or a few scents [37] , thus, the presence of a higher number of ORs may indicate greater diversity in odour sensing. To investigate the types and numbers of ORs in species with different features, ORs from seven species ( G. japonicus , X. tropicalis , D. rerio , An. carolinensis , H. sapiens , Al. sinensis and T. rubripes ) were compared. Because the assembly of ORs is difficult, then the assembly quality of these genomes is a notable concern for the comparative analysis of ORs. The parameters associated with the genome assembly quality are listed in Supplementary Table 24 . The comparative results show that the number of OR genes in G. japonicus (251) is almost three times that in A. carolinensis , a diurnal relative of G. japonicus (87) ( Fig. 5 , Supplementary Table 25 ). Furthermore, nocturnal G. japonicus had many functional γ-ORs for detecting airborne chemicals, which may serve to complement visual senses when seeking prey [33] , [38] . The ability to detect airborne chemicals has been shown to contribute to survival in nocturnal lizards and birds [38] , [39] . Likewise, the substantial expansion of OR genes for scenting airborne odorants in geckos might improve their nighttime survival. 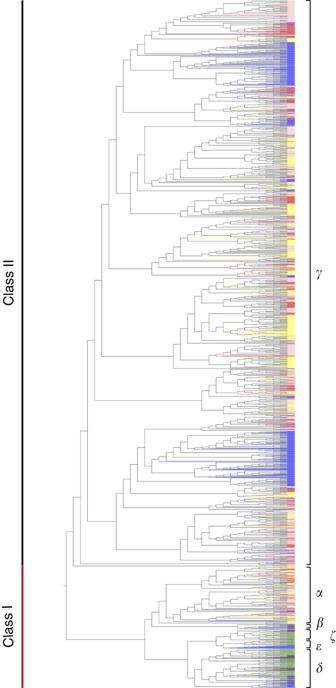Figure 5: Phylogenetic tree of functionalORgenes in seven species. The Class I genes (includingα,β,ɛ,ζandδ ORs) encode proteins used for scent detection in water. The Class II gene (γ-OR) encode proteins used for scent detectionin air.G. japonicushas undergone extensive expansion in Class II genes. Red,G. japonicus; blue,X. tropicalis; green,D. rerio; purple,An. carolinensis; yellow,H. sapiens; pink,Al. sinensis; black,T. rubripes. Figure 5: Phylogenetic tree of functional OR genes in seven species. The Class I genes (including α , β , ɛ , ζ and δ OR s) encode proteins used for scent detection in water. The Class II gene ( γ - OR ) encode proteins used for scent detectionin air. G. japonicus has undergone extensive expansion in Class II genes. Red, G. japonicus ; blue, X. tropicalis ; green, D. rerio ; purple, An. carolinensis ; yellow, H. sapiens ; pink, Al. sinensis ; black, T. rubripes . Full size image Positive selection for tail regeneration in G. japonicus Geckos can detach their tails when they are attacked, and this adaptive physiological process has evolved in many saurian animals to enable quick escape from predators. On tail detachment, multiple tissue regeneration pathways initiate some conserved repair processes including wound healing [40] , blastema formation and tissue remodelling [41] , [42] , [43] . Following this, a new tail will grow within a few months. We searched the G. japonicus genome for genomic regions showing positive selection for tail regeneration in G. japonicus , as such genes are likely important to this process. To identify PSGs, single-copy orthologs were selected from six reptile gene families ( G. japonicus , An. carolinensis , Al. sinensis , C. mydas , Pelodiscus sinensis and P. bivittatus ). Then, we carried out multiple alignments of the single-copy orthologs and calculated the Ka/Ks ratios to identify PSGs in three reptile species ( G. japonicus and An. carolinensis two species with tail regeneration ability, as well as Al. sinensis , a species without this ability). We obtained 155, 178 and 171 PSGs from G. japonicus , An. carolinensis and Al. sinensis , respectively ( Supplementary Table 26 ). Gene Ontology annotation revealed that some PSGs of G. japonicus were likely related to regenerative abilities, as these PSGs were enriched in the categories of wound healing, tissue regeneration, cell proliferation or migration, prostaglandin biosynthetic process and other relevant categories ( Fig. 6a ). These biological processes are essential for successful regeneration, as reported by many studies on limb and tail regeneration in other species [40] , [41] , [42] , [43] , [44] . The PSGs in A. carolinensis and G. japonicus contain several shared Gene Ontology terms, such as cell proliferation and prostaglandin biosynthetic process. It is notable that prostacyclin synthase ( PTGIS ) and prostaglandin–endoperoxide synthase 1 ( PTGS1 ), which are involved in prostaglandin biosynthesis, were under positive selection in both G. japonicus and A. carolinensis. This indicates the likelihood that these genes are involved in similar biological processes that may promote tail regeneration after injury. To investigate whether the PSGs in G. japonicus had activity during tail regeneration, we collected transcriptome data from regenerating stump tissue at different time points following tail amputation. The results showed that 69% of the PSGs were upregulated at 1 day, 3 days or 7 days after autotomy ( Fig. 6b ). Among these genes, the expression of both PTGIS and PTGS1 , which encode key enzymes in prostaglandin synthesis, increased by 3 days after tail amputation. Prostanoids have been reported to be involved in the regeneration of various tissues and organs, including liver, muscle, nerve and tail in different species [45] , [46] , [47] , [48] ( Fig. 6c ). These findings support the hypothesis that PSGs may be involved in tail regeneration or other adaptive physiological processes in G. japonicus. 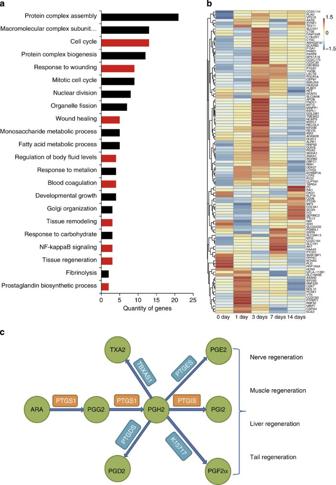Figure 6: Positively selected genes (PSGs) related to tail regeneration inG. japonicus. (a) Analysis of 155 PSGs inG. japonicusbased on representative gene ontology biological processes. Categories with red bars such as cell cycle (GO:0007049), response to wounding (GO:0009611), wound healing (GO:0042060), tissue regeneration (GO:0042246), tissue remodelling (GO:0048771), blood coagulation (GO:0007596) and prostaglandin biosynthetic process (GO:0001516) are likely to be involved in tail regeneration after autotomy. (b) Heatmap of 107 PSGs inG. japonicusat different time points following tail autotomy. Approximately 70% of the PSGs were detected in transcriptome data. (c) Pathway of arachidonic acid (ARA) metabolism inG. japonicus. The circles with green backgrounds represent ARA and its derivatives. The boxes with orange backgrounds show the key synthases under positive selection inG. japonicusgenome. The boxes with blue backgrounds show the normal synthases inG. japonicusgenome. Figure 6: Positively selected genes (PSGs) related to tail regeneration in G. japonicus . ( a ) Analysis of 155 PSGs in G. japonicus based on representative gene ontology biological processes. Categories with red bars such as cell cycle (GO:0007049), response to wounding (GO:0009611), wound healing (GO:0042060), tissue regeneration (GO:0042246), tissue remodelling (GO:0048771), blood coagulation (GO:0007596) and prostaglandin biosynthetic process (GO:0001516) are likely to be involved in tail regeneration after autotomy. ( b ) Heatmap of 107 PSGs in G. japonicus at different time points following tail autotomy. Approximately 70% of the PSGs were detected in transcriptome data. ( c ) Pathway of arachidonic acid (ARA) metabolism in G. japonicus . The circles with green backgrounds represent ARA and its derivatives. The boxes with orange backgrounds show the key synthases under positive selection in G. japonicus genome. The boxes with blue backgrounds show the normal synthases in G. japonicus genome. Full size image Gecko is an important clade of reptile that possesses several amazing abilities, such as the ability to cling at vertical surface and tail regeneration. These characteristics have been extensively investigated for many years. However, the absence of genomic data for Gekkonidae species hinders the mechanism study underlying these interesting phenomena. In this study we acquired the genome sequence of G. japonicus and used this information to investigate the genetic basis of many behavioural and physiological characteristics of geckos by searching for key genes potentially involved in clinging ability, low-light visual activity, highly developed olfaction and regenerative ability. Although our study cannot be considered as an in-depth analysis at the present stage, it provides a foundation for future mechanistic studies, particularly with regard to regeneration. We identified potential candidate genes that might contribute to the regeneration process using genome comparative analysis. Such candidates include PTGIS and PTGS1 , which are involved in prostaglandin synthesis. Prostaglandin metabolism was recently reported to be tightly associated with regeneration in multiple tissues [49] . The timing and manner of the involvement of these genes in tail regeneration of G. japonicus is an attractive topic for further study. In addition, gecko species can also serve as an important model for the studies of sex determination [50] and reproductive strategies [51] , for the reasons that these species situate on the nodes switching environment sex determination to genetic sex determination, oviparity pattern to viviparity pattern. The G. japonicus genomic data obtained in the current study will be of great value in studying these essential evolutionary events. G. japonicus sample The G. japonicus used in this study were sampled in Jiangsu, China. The adult geckos were freely fed mealworms and given water during the whole experiment. All experimental protocols pertinent to animals were given before approval by the Laboratory Animal Care and Use Committee of the Nantong University. Genome sequencing and assembly Genomic DNA was extracted from tissues of an adult male G. japonicus . The DNA was fragmented and the fragments were purified by electrophoresis for whole-genome sequencing. DNA Libraries were constructed according to the ‘ Mate Pair Library v2 Sample Preparation Guide for 2 – 5 kb Libraries ’ and ‘ Paired-End Sample Preparation Guide ’ from Illumina. PCR amplification was performed following the addition of adaptors, and the products were clustered for the mate-pair libraries (insert size ≥2 Kb). The genomic DNA was sequenced using Illumina Hiseq2000 (20 lanes, 330.90 Gb, 131.35 × ). Raw data were generated, after filtering 233.49 Gb of clean data remained for de novo assembly. Whole-genome assembly was performed using SOAPdenovo [52] and SSPACE software [53] . Furthermore, 10 fosmid clones were subjected to Sanger sequencing and were used as reference data to ensure genomic coverage. Genome annotation and evolution Repeats in DNA sequence of G. japonicus were characterized by homologue-based identification using RepeatMasker ( http://www.repeatmasker.org ) and Repbase [54] . Repeated proteins were marked using RepeatProteinMask( http://www.repeatmasker.org ), and de novo interspersed repeat annotation was performed using RepeatModeler ( http://www.repeatmasker.org/RepeatModeler.html ). An extra RepeatMasker analysis was applied after de novo identifications of repeats. In addition, tandem repeats were identified using Tandem Repeat Finder [55] . Gene prediction was created by GLEAN ( http://sourceforge.net/projects/glean-gene ) integration of de novo and homologous gene models. RNA-seq data were subsequently used to refine the gene set. De novo prediction was performed based on the repeat-masked genome. Two programs AUGUSTUS [56] and GENSCAN [57] were applied in the prediction. The homologue-based prediction included the mapping of protein sequences (downloaded from NCBI) of closely related representative species An. carolinensis , Gallus gallus , Homo sapiens , Meleagris gallopavo and Xenopus tropicalis to the genome using TblastN, aligning and searching for accurate spliced alignments using GeneWise [58] . The EST of G. japonicus (downloaded from NCBI) was aligned against the assembled genome using BLAT to generate spliced alignments, and PASA was used to filter the overlapping sequences to link the spliced alignments and predict the possible gene model. Evidences were integrated by GLEAN to produce a consensus gene set. In addition, transcriptomes of multiple tissues were aligned to the genome using TopHat [59] . These were assembled using Cufflinks [60] to improve the accuracy and completeness of the predicted gene set. To conclude gene functions, we scanned the final gene set with KEGG [61] , SwissProtand TrEMBL [62] . InterProScan was also used to confirm motifs and domains in the final gene set of G. japonicus [63] . Gene family expansion We identified gene family expansion and contraction using CAFÉ [64] , which employed a random birth and death model to study gene gain and loss in gene families across a user-specified phylogeny. The global parameter λ , which described both the gene birth ( λ ) and death ( μ =− λ ) rate across all branches in the tree for all gene families, was estimated using maximum likelihood. A conditional P value was calculated for each gene family, and families with conditional P values less than threshold (0.0001) were considered to have accelerated rates of gain or loss. We identified branches that were responsible for low overall P values of significant families. Phylogenetic analyses We constructed a phylogenetic tree that included Alligator sinensis , Anolis carolinensis , Pelodiscus sinensis , Chelonia mydas , Xenopus tropicalis , Canis familiaris , Oryzias latipes , Homo sapiens , Meleagris gallopavo , Gallus gallus , Ornithorhynchus anatinus , Danio rerio , Taeniopygia guttata , Python molurus bivittatus and G. japonicus using 696 single-copy orthologous genes from gene family construction. Each of the orthologous genes was subjected to multiple sequence alignment with Muscle [65] and concatenated into a super sequence. PhyML [66] was used to construct the phylogenetic tree under the GTR and Inv-γ model functions. The same sequence set was applied to estimate the periods of species divergence using the program PAML MCMCTREE under correlated molecular clock function in the approximate likelihood calculation method [67] . The correlated molecular clock and REV substitution model were selected to perform estimation. The MCMC process of PAML mcmctree was run to sample 100,000 times with a sample frequency of 50, after a burn-in of 5,000,000 iterations. Fossil calibrates were derived from http://www.fossilrecord.net/dateaclade/index.html . Positively selected genes We calculated Ka/Ks ratios for all single-copy orthologs of G. japonicus , Anolis carolinensis , Alligator sinensis , Python molurus bivittatus , Chelonia mydas and Pelodiscus sinensis. Alignment quality was essential for estimating positive selection. Thus, orthologous genes were first aligned using PRANK [68] , a favored alignment tool for molecular evolution studies [69] . We used Gblocks to remove ambiguously aligned blocks within the PRANK alignments [70] . We employed ‘codeml’ in the PAML package with the free-ratio model to estimate Ka, Ks and Ka/Ks ratios on different branches. The differences in the mean Ka/Ks ratios for single-copy genes between G. japonicus and each of the other species were compared with paired Wilcoxon rank-sum tests. After filtering out the false positive, we obtained a final total of 155 positive selection genes in G . japonicus . Accession codes: This Whole Genome Shotgun project of Gekko japonicus has been deposited at DDBJ/EMBL/GenBank under the accession LNDG00000000 . The version described in this paper is version LNDG01000000 . The RNA-Seq data of Gekko japonicus have been deposited in NCBI database under the accession code SRA304902. How to cite this article: Liu, Y. et al. Gekko japonicus genome reveals evolution of adhesive toe pads and tail regeneration. Nat. Commun. 6:10033 doi: 10.1038/ncomms10033 (2015).